Metabolic properties in stroked rats revealed by relaxation-enhanced magnetic resonance spectroscopy at ultrahigh fields 1 H magnetic resonance spectroscopy (MRS) yields site-specific signatures that directly report metabolic concentrations, biochemistry and kinetics—provided spectral sensitivity and quality are sufficient. Here, an enabling relaxation-enhanced (RE) MRS approach is demonstrated that by combining highly selective spectral excitations with operation at very high magnetic fields, delivers spectra exhibiting signal-to-noise ratios >50:1 in under 6 s for ~5 × 5 × 5 (mm) 3 voxels, with flat baselines and no interference from water. With this spectral quality, MRS was used to interrogate a number of metabolic properties in stroked rat models. Metabolic confinements imposed by randomly oriented micro-architectures were detected and found to change upon ischaemia; intensities of downfield resonances were found to be selectively altered in stroked hemispheres; and longitudinal relaxation time of lactic acid was found to increase by over 50% its control value as early as 3-h post ischaemia, paralleling the onset of cytotoxic oedema. These results demonstrate potential of 1 H MRS at ultrahigh fields. Magnetic resonance imaging (MRI) is indispensable for understanding the biology of healthy tissues [1] , [2] as well as for non-invasively diagnosing disease [3] , [4] . MRI delivers valuable spatially resolved insight despite its primary focus on a single molecule: the water residing within tissues. Central to this achievement are the diverse physical interactions that will affect the magnetic resonance (MR) signal of water; foremost among them are the contrast mechanisms that, based on morphology, function and disease, modulate spin–lattice and spin–spin ( T 1 and T 2 ) relaxation times, as well as its diffusivity and hydrogen exchanges [5] , [6] . Despite this valuable and varied source of contrast mechanisms many of the properties reflected by water remain ambiguous, challenging the biological interpretation of these changing MR parameters. In stroke, for example, increases in diffusion-weighted MRI signals of water are clear reporters on the early onset of an infarct [7] , yet the structural changes underlying these signal changes remain the subject of vigorous investigations [8] , [9] . Clearly, a much richer information about physiology, microstructure and function, would arise if MR measurements were to shift from ‘the solvent’ to the numerous small molecules that are actually involved in the biological functions. For central nervous system (CNS) studies, in particular, endogenous metabolites could report on crucial events such as neurotransmission, pH, redox states, membrane synthesis and energetic turnover [10] , [11] . Metabolites could also serve as early reporters for neurological disorders such as dementia, schizophrenia, and Parkinson’s and Huntington’s diseases [12] , about the fate of malignancies [13] , and about ischaemic processes [7] . Magnetic resonance spectroscopy (MRS) is an ideal methodology to investigate these CNS metabolic aspects in vivo and noninvasively [14] . Whereas MRI contrasts delineate anatomical landmarks based on single resonance of water, MRS seeks to resolve the frequency signatures associated with various endogenous metabolites via their chemical shifts [14] , [15] . MRS thus can report about neurotransmitters (glutamate, aspartate and γ-aminobutyric acid), bioenergetic metabolites (creatines (Cre), lactic acid (Lac)) and osmolytes (N-acetyl-asparate (NAA)), molecules involved with membrane synthesis (cholines (Cho)), sugars (glucose, inositols) and other CNS metabolites present at millimolar concentrations [14] , [15] . MRS has afforded valuable insights into the nature of disease metabolism [16] , [17] , [18] ; furthermore, since some of these metabolites are selectively compartmentalized, for example, NAA is considered intraneuronal, whereas myo-inositols reside mostly in astrocytes, MRS can potentially resolve structurally distinct cellular environs. Despite all this potential, most MRS measurements are limited to depicting in vivo relative concentrations of various metabolites. This is particularly restrictive when considering the wealth of information that water-based MRI successfully delivers by exploiting relaxation, diffusion and other contrast mechanisms. Indeed, complementing information about metabolic concentrations —or even metabolic density maps—with 1 H MR’s many other potential sources of contrast could provide a much richer information about a tissue under investigation. The current restricted versatility of MRS does not reflect an intrinsic limitation but is rather a consequence of (i) the need to suppress the ~10,000 times stronger water resonance to enable the observation of millimolar-level metabolites, a process that often creates spectral distortions hindering complex MRS measurements; and (ii) the limited sensitivity associated with the observation of low-concentration endogenous metabolites that a priori precludes rapid experiments and, hence, the execution of more complex and time-consuming MRS sequences. These two factors conspire to render the relaxation- and diffusion-based probing of metabolites under in vivo conditions [19] , [20] , [21] , [22] , [23] , [24] a considerable challenge. In this study, we present and demonstrate a general MRS approach that enables high-fidelity measurements of relaxation, diffusion and kinetic interactions of metabolites within healthy and diseased tissues. The method yields 1 H MRS with high signal-to-noise ratio (SNR) per unit time by harnessing two complementary features: the use of a non-water-suppressed sequence [25] that benefits from an enhanced relaxation arising from selective frequency excitation [26] , and the execution of these experiments at ultrahigh magnetic fields for which 1 H MRS is greatly facilitated by polarization, spectral and—foremost—relaxation characteristics. Sensitized in this fashion, the duration of localized in vivo MRS measurements can be remarkably reduced, enabling the observation of novel, metabolite-specific behaviours based on restricted diffusion, relaxation and exchange. This potential is demonstrated with an array of ‘firsts’ in CNS spectroscopy in animal models of unilateral stroke, including SNRs exceeding 50:1 from 6-s in vivo recordings, the observation of differential metabolic diffusive confinements in disordered anisotropic tissue microstructures and new metabolic fingerprints of stroke arising from spectral regions located downfield of the water resonance. Finally, relaxation-based 1 H MRS measurements were used to probe differential interactions of various metabolites upon stroke, suggesting changing microscopic environments and macromolecular bindings. Overall, this strategy facilitates the study of relationships between the microstructure of the brain, metabolism and interactions of endogenous metabolites with their host tissues. Numerous extensions of this potential to other CNS diseases and to other biological tissues, can be envisioned. Features of ultrahigh-field relaxation-enhanced 1 H MRS The relaxation-enhanced (RE) MRS methodology hereby employed, relies on an excitation-contrast-localization-acquisition layout ( Fig. 1 ). While numerous variants of this scheme can be conceived, a key common element is the avoidance of long-term perturbations of water or macromolecular resonances based on a RE strategy [25] . In RE MRS, the data are collected using a highly spectrally selective spin echo sequence targeting only the resonances of interest; for instance, the methyl peaks of Lac, NAA, Cre and Cho. In the absence of pre-saturation or crushing, this selectivity ensures that the bulk of both the water and macromolecular reservoirs remain largely unperturbed, benefiting the excited spins by minimizing potential magnetization transfer processes driven by cross-relaxation from surrounding protons, and/or facilitating a fast recovery driven by chemical exchanges between labile 1 Hs and water [26] . Selectively excited metabolic resonances can then be subjected to a variety of contrast mechanisms that sensitize them to their environments. In this study filters were applied that monitored the responses of metabolites to restricted diffusion and tissue micro-architectures, that used spectral profiles tailored to directly observe the labile protons resonating downfield of water, and that incorporated various relaxation-monitoring delays to measure the dynamic properties of metabolites. For all filters, the chemical shift evolution accrued during the initial excitation is refocused with frequency-selective pulses so as to ensure high-quality 1 H lineshapes. With these selective contrasts imposed, the targeted metabolites are spatially localized using a fully refocused module confining the observable magnetization to a volume of interest, and signals are finally acquired with a spectroscopic or spectroscopic imaging module ( Fig. 1 ). 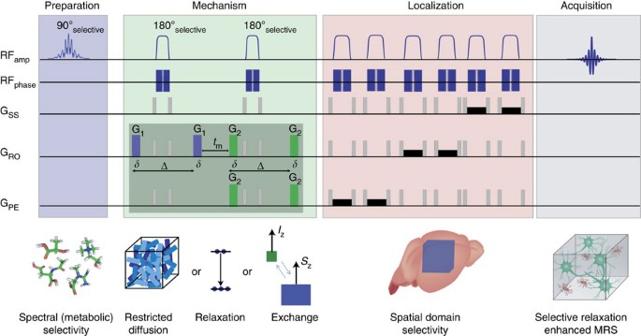Figure 1: General layout of relaxation-enhanced (RE) spin–echo1H MRS. The approach encompasses a spectrally selective excitation perturbing only the resonances of interest, a contrast mechanism module probing metabolic interactions with host tissues—whether via restricted diffusion (illustrated here with a sequence aimed at probing highly heterogeneous microarchitectural features in the shaded region), relaxation or magnetization exchange with macromolecules, a localization by adiabatic selective refocusing (LASER) sequence48imparting spatial selectivity, and a signal acquisition based on either spectroscopic or spectroscopic imaging methods. Gss, slice selective gradients; GRO, readout gradients; GPE, phase encoding gradients; RF, radiofrequency- and acquisition-related manipulations. Figure 1: General layout of relaxation-enhanced (RE) spin–echo 1 H MRS. The approach encompasses a spectrally selective excitation perturbing only the resonances of interest, a contrast mechanism module probing metabolic interactions with host tissues—whether via restricted diffusion (illustrated here with a sequence aimed at probing highly heterogeneous microarchitectural features in the shaded region), relaxation or magnetization exchange with macromolecules, a localization by adiabatic selective refocusing (LASER) sequence [48] imparting spatial selectivity, and a signal acquisition based on either spectroscopic or spectroscopic imaging methods. G ss , slice selective gradients; G RO , readout gradients; G PE , phase encoding gradients; RF, radiofrequency- and acquisition-related manipulations. Full size image This strategy leads to spatially localized spectra, reflecting the contrasts imposed with a very high sensitivity ( Fig. 2 ). In vivo 1 H MRS acquired in only 6 s (eight scans) from a 5 × 5 × 5 (mm) 3 rat brain voxel at 21.1 T (900 MHz 1 H frequency) showed a SNR >50:1 for the NAA peak (with a SNR >10:1 and a clean baseline observed in only one scan), and a nearly complete absence of the water resonance without any form of active suppression ( Fig. 2a ). Besides the natural increase in sensitivity afforded by a 21.1 T magnet, inherent factors contributing to the high SNR and high signal-to-artefact ratios observed for these MR spectra pertain to the relaxation times arising at these ultrahigh fields. At 21.1 T, T 2 relaxation times are nearly an order of magnitude longer for the metabolites than for their water 1 H counterparts, while metabolic T 1 times are ~2–3 times shorter than those of water. These favourable parameters, along with the power dependence of SNR on B 0 , are exploited by the RE strategy to obtain the clean metabolic spectra and flat MRS baselines shown in Fig. 2a . 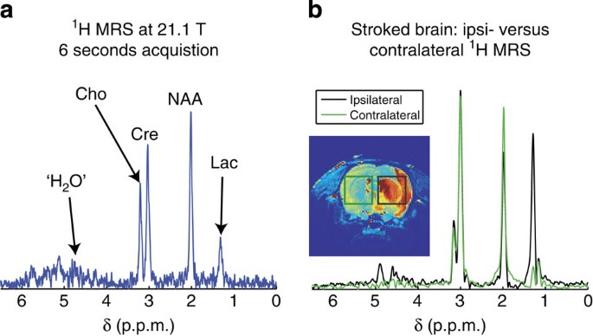Figure 2: Spectral quality arising from RE1H MRS at ultrahigh fields. (a) Prototypical1H MR spectrum recorded in 6 s from a 125-μl voxel centred in a stroked hemisphere of a representativein vivorat brain (N=6). The signal-to-noise ratio (SNR) of NAA exceeds 50:1, and little remains of the water resonance despite being ~10,000 times stronger than the metabolic signals. (b) Spectra acquired in ~5 min from the ipsi- and contralateral hemispheres of a (different) stroked rat, with indicated squares placed within the inset anatomical1H MR image representing the voxels acquired. Figure 2b displays RE 1 H MRS spectra recorded in 5 min from identical voxels centred in the ipsi- and contralateral hemispheres of a stroked rat, 24-h post ischaemia. The expected increase in Lac and decrease in NAA resonance intensities are readily observed, with the SNR for NAA in the contralateral hemisphere approaching 300. Notice as well that despite its J-coupling, Lac’s methyl resonance appears well phased; this stems from the high spectral selectivity of the sequence which, by not inverting Lac’s methyl coupling partner, performs a sort of homonuclear J-echo. With this good sensitivity and spectral fidelity as a starting point, more elaborate MRS schemes can be conducted as illustrated below. Figure 2: Spectral quality arising from RE 1 H MRS at ultrahigh fields. ( a ) Prototypical 1 H MR spectrum recorded in 6 s from a 125-μl voxel centred in a stroked hemisphere of a representative in vivo rat brain ( N=6 ). The signal-to-noise ratio (SNR) of NAA exceeds 50:1, and little remains of the water resonance despite being ~10,000 times stronger than the metabolic signals. ( b ) Spectra acquired in ~5 min from the ipsi- and contralateral hemispheres of a (different) stroked rat, with indicated squares placed within the inset anatomical 1 H MR image representing the voxels acquired. Full size image Metabolic confinements monitored in vivo upon ischaemia Diffusion-weighted MRI has a central role in the early diagnosis and prognosis of stroke [7] , [27] , [28] , yet the determinants underlying diffusivity variations of water post ischaemia are still not fully understood [9] , [29] . The nonspecific nature of water-based MRI measurements prevents the selective probing of distinct cellular morphologies. By contrast, metabolites can exhibit a selective compartamentalization [30] , and extending diffusion measurements to metabolic resonances could crucially improve the specificity of the measurements towards different neural tissue elements [18] , [20] , [31] , [32] , [33] , [34] , [35] . One of the goals of this study was to explore the potential of in vivo RE MRS to detect the underlying micro-architectures to which selected metabolites are confined in healthy and stroked hemispheres. To this end, we focused on angular double-pulsed field gradient (dPFG) experiments [36] (shaded box under ‘Filter’ in Fig. 1 )—a challenging measurement that within the context of CNS studies has so far been performed only on the abundant water signals. dPFG correlates random molecular displacements by applying pairs of diffusion-sensitizing gradients G 1 and G 2 whose relative angle ψ is varied. When restricted diffusion occurs, this kind of correlation can probe local restrictions via characteristic signal amplitude modulations [36] , [37] , [38] , whose angular dependency can be used to extract microarchitectural features even in highly heterogeneous scenarios—for instance, when compartments are randomly oriented [38] . To study the kind of restricted diffusion that metabolites may experience in randomly oriented brain microstructures in health and in disease, dPFG RE 1 H MRS experiments were conducted in rats that had been subject to a transient, 1.5-h middle cerebral artery occlusion (MCAO) to produce a severe unilateral ischaemia ( Fig. 3 , upper inset). dPFG 1 H MRS spectra arising from signals localized on the contra- and ipsilateral MCAO hemispheres were recorded 24-h post ischaemia, by varying the angle ψ between G 1 and G 2 . Despite the complexity and signal losses associated with the angular dPFG experiment, whose successful in vivo execution even on the strong water signals upon stroke is yet to be achieved, high-fidelity data from the metabolites of interest were obtained ( Fig. 3a,b ). Notice the negligible residual water signal, the absence of baseline distortions and the short acquisition times (~4 min) that characterize these spectra—for which the SNR of NAA in the contralateral hemisphere reached ~250 for ψ =0°. The cos(2 ψ )-like modulations arising from these data ( Fig. 3c,d ) reflect the diffusion mode of these metabolites, representing the first unequivocal evidence for restricted metabolic diffusion in the randomly oriented compartments of an in vivo brain. The local anisotropies of the otherwise randomly oriented structures leading to these oscillations can be described by apparent L/R eccentricity ratios, where L is a cylinder’s long axis and R is its radius. [37] Fits of these data under the assumption of fully restricted diffusion, reveal that Lac, NAA, Cre and Cho eccentricities in the contralateral hemisphere are 9.7±2.0, 11.2±0.9, 10.6±0.9 and 11.1±0.8, whereas in the ipsilateral hemisphere these increase to 11.9±0.9, 12.7±0.8, 12.5±0.6 and 12.1±0.9, respectively. When similar spectra were quantified across rats, a statistically significant increase in eccentricity was observed 24 h after the onset of ischaemia for NAA, Cre and Cho ( P <0.05, N=6 , one-way analysis of variance, Fisher means comparison); interestingly, this statistical analysis finds Lac diffusing in consistently less eccentric spaces compared with NAA ( P <0.05, one-way analysis of variance, Fisher means comparison), which is considered an intraneuronal marker. Because the dPFG amplitude modulations reflect local eccentricities, this difference highlights a genuine confinement of Lac to more spherical environments, presumably reflecting a preferential accumulation of Lac in intracellular—environments. It should be noted that the long echo time (TE) of the sequence inherently weights dPFG experiments towards long T 2 species; however, as metabolic T 2 s are in any case naturally longer than their water counterparts, this provides ample time for diffusing metabolites to probe the morphology in which they are confined. Findings such as these highlight the potential specificity enhancement entailed by probing metabolites that are often confined to specific tissues or cells (such as NAA in neurons and myo-inositol in astrocytes) rather than global water signals. 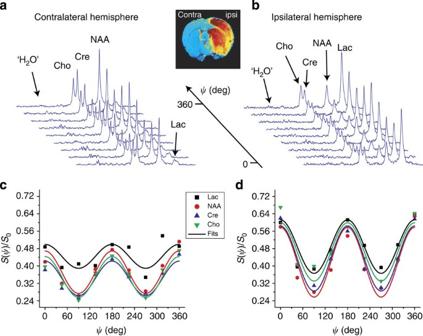Figure 3: Probing microarchitectural features byin vivodPFG RE MRS. (a,b)1H spectra arising from contra- and ipsilateral hemispheres of a representative rat (out ofN=6) subject to unilateral stroke, monitored 24 h post ischaemia. Notice the evident oscillations of the peaks upon varyingψ, which are the hallmark of restricted diffusion in non-spherical, randomly oriented compartments. Further details on these experiments are given in Methods section. (c,d) Peak oscillations observed in panelsa,b, plotted as the ratios between the observed dPFGS(ψ) signals over their non-dPFG resonance intensities versus the inter-gradient angleψ. Notice the clear increase in eccentricity in the stroked region revealing an enhancement in the anisotropic structures in the micrometre scale, as well as the less eccentric confinement of lactate suggesting its differential compartmentalization. Figure 3: Probing microarchitectural features by in vivo dPFG RE MRS. ( a , b ) 1 H spectra arising from contra- and ipsilateral hemispheres of a representative rat (out of N=6 ) subject to unilateral stroke, monitored 24 h post ischaemia. Notice the evident oscillations of the peaks upon varying ψ , which are the hallmark of restricted diffusion in non-spherical, randomly oriented compartments. Further details on these experiments are given in Methods section. ( c , d ) Peak oscillations observed in panels a , b , plotted as the ratios between the observed dPFG S ( ψ ) signals over their non-dPFG resonance intensities versus the inter-gradient angle ψ . Notice the clear increase in eccentricity in the stroked region revealing an enhancement in the anisotropic structures in the micrometre scale, as well as the less eccentric confinement of lactate suggesting its differential compartmentalization. Full size image Downfield 1 H resonances as potential stroke biomarkers Nearly all metabolic MRS studies performed in vivo within the context of CNS disorders have hitherto focused on the spectral region upfield of water where aliphatic protons resonate [14] , [15] . The spectral region positioned downfield of water (5–10 p.p.m.) has been probed only rarely in healthy tissues [39] , [40] or in the context of disease [41] , most likely because this region contains labile protons whose exchange with water renders them hard to detect upon using conventional, active solvent suppression. This downfield spectral region contains important resonances including ATP, glutamine, glutamate, gluthatione, homocarnosine, imidazole, NAD + , phenylalanine, phosphocreatine, tryptophane and tyrosine [42] , whose direct characterization could open new vistas in understanding CNS metabolism. To test whether the approach in Fig. 1 is suitable for downfield evaluations, in vivo experiments were performed with an excitation involving a single band targeting the 5.7–9.7 p.p.m. region and exhibiting a ≤0.06° pulse angle excitation at the 4.75-p.p.m. water frequency. Spectra resulting from ipsi- and contralateral hemispheres of a stroked rat 24-h post ischaemia collected in only 10 min reveal at least nine resolved resonances ( Fig. 4 ). Out of these, NAA can be unambiguously assigned, yet the origin of the other peaks remains to be fully identified [39] , [40] , [42] . The potential of these peaks as stroke biomarkers is also evident in Fig. 4 : peaks labelled ‘ a’, ‘c’ and ‘h’ are either unaffected by the ischaemic process or promptly recover from it, whereas all remaining peaks show varying decreases in their amplitudes. Assuming that the assignments provided in vitro [43] apply also in vivo , peaks ‘a’ and ‘ c ’ could potentially represent hydroxyl moieties of glucose or glucose-6-phosphate, which would imply that, by 24-h post ischaemia, glucose levels are restored in brain tissue by reperfusion. Also, assuming that the peak at ~8.3 p.p.m. reflects the adenosine moiety ATP (one of the few abundant metabolites resonating at such high p.p.m. values [42] ), the decrease shown by ‘ i’ in Fig. 4 suggests a significant impairment of the energetic cycle. It is overall clear that, pending their full assignment, the differential behaviours observed for the numerous peaks now resolved in the downfield region can provide valuable insight to diagnose and evaluate stroke. 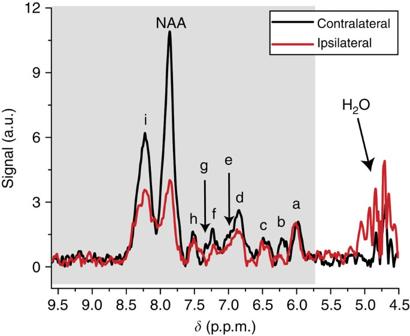Figure 4: Stroke biomarking based on RE1H MRS of downfield resonances. Spectra arising upon exciting the spectral region downfield from water (shaded region) in a representative stroked rat (out ofN=2) after 10 min of signal averaging the sequence inFig. 1with a TE of ~60 ms. Some of these peaks remain unaffected by or have recovered from the initial stroke at this 24-h post-MCAO time point, whereas other resonances are significantly affected by the ischaemia. Figure 4: Stroke biomarking based on RE 1 H MRS of downfield resonances. Spectra arising upon exciting the spectral region downfield from water (shaded region) in a representative stroked rat (out of N= 2) after 10 min of signal averaging the sequence in Fig. 1 with a TE of ~60 ms. Some of these peaks remain unaffected by or have recovered from the initial stroke at this 24-h post-MCAO time point, whereas other resonances are significantly affected by the ischaemia. Full size image Metabolic interactions with endogenous macromolecules Additional valuable targets for metabolic characterizations rest in the spin relaxation times, which could be diagnostic reporters on the binding of metabolites to larger macromolecular structures or probes of compartmentalization. Although considerable efforts have been invested in assessing these relaxation times [19] , [21] , [22] , including in the context of CNS disease [44] , these measurements are still challenged by the need to optimize water suppression and by limited sensitivity. Here, we utilized the RE MRS approach to measure the post-stroke T 1 s of Lac, Cho, Cre and NAA in vivo upon applying a progressive saturation filter [21] . 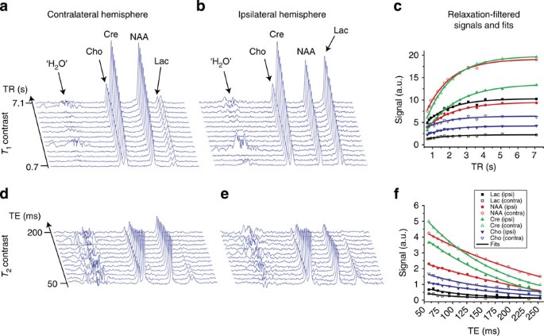Figure 5: Probing metabolic relaxation times on stroked ratsin vivo. (a–c) MRS progressive saturation curves recorded from a representative rat (out ofN=6studied) using the scheme inFig. 1on 125 μl voxels 3-h post ischaemia, leading to a robust quantification of metabolicT1s (solid lines inc) in under 30 min (with NA=48 scans per point). (d–f) MetabolicT2s 24-h post ischaemia acquired from a 125-μl voxel in a representative rat (out ofN=4 studied); these measurements took 16 scans per point and <25 min to acquire overall. Figure 5a,b shows data collected 3-h post ischaemia from the contra- and ipsilateral hemispheres of a representative animal, respectively. The expected exponential buildup of metabolic signals with increasing repetition time (TR) is readily observed for all resonances of interest, with a high SNR that yields the entire measurement—comprising 15 points–in under 30 min. Despite the fact that NAA is considered a neuronal viability marker whose concentration has been shown to vary considerably post stroke [23] , data from N =6 rats revealed that NAA T 1 s remains unchanged by the onset of ischaemia , in agreement with a previous lower field study [19] . By contrast, the Lac signal shows a ~50% increase from a contralateral value to in the ipsilateral hemisphere at the very early time point of 3-h post ischaemia ( P <0.05). This increase in apparent T 1 suggests that lactate weakens its average interactions with the macromolecular structures in the host tissue. Cre and Cho , on the other hand, exhibit only minor T 1 changes 3-h post ischaemia, remaining statistically unchanged in both hemispheres upon stroke. Figure 5d–f illustrates analogous experiments for a representative rat, but focusing on metabolic T 2 s at 24-h post ischaemia. These relaxation data show (a) long T 2 s in the range of 100–170 ms for all metabolites, values that could be somewhat biased towards longer T 2 species owing to the long TEs explored, and (b) consistently slower decays in the ipsilateral hemisphere, indicating again weaker interactions between metabolites and macromolecules within host tissues upon stroke. Notably, the relatively long T 2 s and short T 1 s of metabolites compared with water at 21.1 T support the benefits of the RE high-field MRS sequence, and open new possibilities for the application of more advanced spectroscopic techniques, such as multi-dimensional spectral and high-definition spatial/spectral acquisitions. Figure 5: Probing metabolic relaxation times on stroked rats in vivo . ( a – c ) MRS progressive saturation curves recorded from a representative rat (out of N=6 studied) using the scheme in Fig. 1 on 125 μl voxels 3-h post ischaemia, leading to a robust quantification of metabolic T 1 s (solid lines in c ) in under 30 min (with NA=48 scans per point). ( d – f ) Metabolic T 2 s 24-h post ischaemia acquired from a 125-μl voxel in a representative rat (out of N= 4 studied); these measurements took 16 scans per point and <25 min to acquire overall. Full size image Probing metabolic interactions within tissues non-invasively and in vivo is a long-standing challenge, particularly when elucidating the intricate relationships between metabolism, structure and function in health and disease [14] , [15] . Contrary to positron emission tomography (PET) or hyperpolarized 13 C MRS, which require injections of radiolabelled tracers or large influxes of slowly relaxing stable isotopes, 1 H MRS utilizes endogenous brain metabolites at physiological concentrations and conditions as molecular reporters. Despite this ideal scenario, MRS is generally limited by the low sensitivity associated with metabolic concentrations. This study sensitizes these measurements by focusing observations to only a few metabolites whose spectral positions are a priori defined and executing selective excitation echo experiments at ultrahigh magnetic fields. A sensitivity synergy then emerges combining the high SNR provided by a state-of-the-art magnet, an optimized radiofrequency coil design, the enhanced field-dependent spectral dispersion that allows one to target the desired metabolites in a very selective manner, cross-relaxation and exchange-induced repolarization effects that arise when leaving the bulk pool of solvent and macromolecular 1 Hs untouched, and an echo sequence whereby any residual water that might have been excited decays before the data acquisition. Particularly valuable to stress are the favourable relaxation properties that arise for performing non-water-suppressed MRS at 21.1 T, with relatively short metabolic T 1 s and long metabolic T 2 s compared with their water 1 H counterparts, facilitating the acquisition of flat baseline spectra. Even if TEs are inherently long, these synergies then result in a very high SNR per unit time and in clean, undistorted baselines; robust spectral features that in turn open avenues of research that have so far eluded MRS. As demonstrated, one such opportunity relied on using diffusion-based dPFG to probe complex metabolic confinements in normal and diseased CNS. When applied to monitor the behaviour of four metabolites, these MR signals unequivocally demonstrated hallmark (yet previously unobserved) signatures for restricted diffusion in randomly oriented, anisotropic structures. Apart from this basic insight, the angular dPFG experiments revealed that Lac diffuses in a different environment than the remaining metabolites. This could help elucidate the nature of conventional diffusion experiments reporting that upon ischaemia water exhibits a decreased diffusivity; in the metabolite-based measurements, this decrease appears to be correlated to increases in the apparent eccentricity of the underlying microstructures. The intriguing stroke- and metabolite-dependent eccentricities revealed by the dPFG experiments warrant further studies to elucidate at a microscopic level the interactions between ischaemic tissues and metabolites, their evolution with recovery and therapies vis-à-vis specific neural tissue elements, as well as their interpretation within the frame of more complex diffusion analytical models [45] . Another objective of this study centred on the spectral resonances appearing downfield from water, which have been notoriously challenging to characterize at lower fields owing to difficulties in avoiding water-suppression schemes. These drawbacks disappear with the application of a sculpted downfield excitation, thereby leading to intense signals that could be measured in under 10 min to provide information that clearly discriminated healthy tissue from diseased. As these downfield resonances represent different metabolites from those conventionally observed containing, for instance, the signatures of ATP and NAD [42] , [46] , such characterizations are expected to provide insights into stroke-related bioenergetics and redox changes. RE MRS also lends itself to efficiently probe metabolic relaxation rates, another set of potential biomarkers for disease and compartmentalization. In this respect it is worth noting that whereas previous studies had reported changes in NAA, Cre and Cho T 1 s beginning around 24-h post ischaemia and associated them to the onset of vasogenic oedema [19] , the sensitivity endowed by RE MRS allowed us to measure increases in Lac’s T 1 as early as 3-h post ischaemia, coinciding with the onset of cytotoxic oedema. In principle, this kind of advantages should also materialize in other tissues as well as for different pathologies. From a physical standpoint, nothing fundamental would prevent these synergies to act as well in ultrahigh-field human brain studies— even if performing such extension would require dealing with the relatively high specific absorption rate exhibited by the localization modules used in the present study. It is worth concluding by reflecting on other new avenues that become accessible by the high SNR offered by RE MRS. These include further relaxation measurements based on Overhauser effects that could aid in peak assignment and in further probing small/macromolecular interactions, saturation-exchange variants that measure solvent accessibility of different sites, multi-dimensional acquisitions based on J couplings to further resolve and assign ambiguous resonances, and additional diffusion-based metabolic measurements. All of these methods require high sensitivity, but are judged compatible with in vivo scanning time scales given the SNR demonstrated in Figs 2 , 3 , 4 , 5 . Another worthy extension includes the realization of accelerated spectroscopic imaging experiments: the fact that the chemical shifts of the targeted metabolites are known a priori implies that selective excitation could be combined with accelerated imaging approaches in order to measure metabolic location with good sensitivity and unprecedented spatial resolutions in reasonable acquisition times. Alternatively, this advancement could open new possibilities for performing in vivo functional MRS and MRSI studies with adequate temporal resolutions. These vistas, as well as further characterizations of health, disease and cellular metabolism based on the present MRS approach, are currently under investigation. All experiments in this study were pre-approved by the Florida State University (FSU) Animal Care and Use Committee (protocol no. 1038), which has been accredited by the Association for Assessment and Accreditation of Laboratory Animal Care, International (AAALAC). FSU is registered as a research facility with the United States Department of Agriculture (registration no. 58-R-0001) and has an Animal Welfare Assurance (no. A3854-01) on file with the US Public Health Service. All animal procedures were performed according to these regulatory bodies and AAALAC guidelines, and every effort was taken to minimize animal suffering, as directed and overseen by a veterinarian who is certified as a specialist in laboratory animal medicine by the American College of Laboratory Animal Medicine. The animals used in this study were juvenile male Sprague–Dawley rats weighing 250 g and age 1.5–2 months at the time of the experiment. The animals were housed in 12 h light/dark cycles. Animal surgery Surgical procedures were performed under aseptic conditions. Ischaemia-reperfusion was achieved by occluding the MCA of juvenile Sprague–Dawley rats for 1.5 h. The animals were anaesthetized with 5% isoflurane and maintained with ~2% isoflurane using a nose cone. A rubber-coated filament (Doccol Corp., Sharon, MA) was guided 1.9 cm through the external carotid artery until the MCA was blocked and blood flow was interrupted to the brain region served by the MCA. Transient occlusion occurred for 1.5 h followed by re-anaesthetization induced again by 5% isoflurane and maintained by 2% isoflurane. The filament was carefully removed to allow reperfusion. Animals were treated to minimize any discomfort and then placed back in their cage for recovery. The same rats were used throughout the experimental time points in this study, including experiments performed both 3- and 24-h post ischaemia. MRI system All experiments in this study were performed with the vertical 21.1-T MRI scanner (11-cm bore size, 6.35-cm gradient bore size) located in the National High Magnetic Field Laboratory Users Facility, operating at a 1 H frequency of 900 MHz and equipped with a Bruker Avance III console (Bruker-Biospin, Billerica, MA). The gradient system used is capable of producing magnetic field gradients of up to 600 mT m −1 in all directions, with a rise time of 120 μs. For both excitation and detection, a home-built quadrature half-saddle coil was used possessing a 33-mm inner diameter, a loaded Q =131 (130 and 132 for each channel), and delivering a ~125-μs hard pulse using ~80 W of peak power). Before experiments, anaesthesia was induced with 5% isoflurane, followed by ~2% for maintenance delivered through a nose cone throughout the MRI scans. The animals were kept at a constant temperature in the MRI scanner by means of gradient chiller temperature and their breathing rate was monitored (SA Instruments, Stonybrook, NY) throughout the experiments and kept at 30–50 breaths per minute. All experiments were respiratory gated. Preparation, refocusing, localization pulses and MRS processing All pulses herein used were derived from the Shinar LeRoux algorithm [47] . For upfield metabolites, an 8-ms polychromatic multiband excitation pulse was designed, targeting only the resonances of interest (Lac, Cre, Cho and NAA). The downfield metabolites shown in Fig. 4 were excited by a single-band 8-ms pulse whose right-most stop band reached ~5.5 p.p.m. Single-band, frequency-swept, quadratic phase refocusing pulses of 4 ms durations, 1.3 kHz B 1max and 4.5 p.p.m. bandwidth were used to refocus chemical shift evolutions accrued during the preparation pulses. The localization was achieved using the 3D-LASER (localization by adiabatic selective refocusing) methodology [48] that entailed the applications of three pairs of adiabatic 5-ms 1.6 kHz B 1max and 20 p.p.m. bandwidth slice-selective refocusing pulses imparting spatial selectivity in all three dimensions, respectively. Under these localization conditions, the maximum shift-driven displacement between the voxels associated to the different metabolites was under 1 mm. Two voxels of interest spanning a 5 × 5 × 5 (mm) 3 volume were then located: one at the core of the ischaemic region and another symmetrically placed in the contralateral hemisphere. The quality of the MRS localization was ascertained by collecting images incorporating identical LASER localization modules. Spectra were processed by subjecting the conventionally averaged time domain signals to zero filling (32 k), apodization with a 25-Hz exponential line broadening, Fourier transform and magnitude calculation. dPFG MRS experiments These restricted diffusion correlation experiments [36] , [37] , [38] , [45] relied on two gradient pairs G 1 and G 2 , of duration δ and separation Δ ( Fig. 1 , shaded filter) separated by a long mixing time ( t m ). The magnitude and direction of G 1 was kept constant, while the relative orientation of the second gradient G 2 varied about the axis subtended by G 1 , that is, the relative angle ψ between the two gradients is the variant in angular dPFG. Localized dPFG MRS experiments were performed in the rat brains 24-h post ischaemia with | G 1 |=| G 2 |=48 G cm −1 , Δ=53.5 ms, δ =2.5 ms and t m =24 ms on a voxel size of 5 × 5 × 5 (mm) 3 placed within the stroke or in the contralateral hemisphere. Each trace was acquired with TR/TE =1,500/187 ms and number of averages (NA)=160, resulting in 4 min of scan time per trace or 36 min for the nine ψ values spanning 0:45:360 degrees. The amplitude modulation for the peaks was quantified by fitting the data to a simple S ( ψ )/ S 0 = A+B(cos(2 ψ )) curve in MATLAB (Mathworks, Nattick, MA), and the amplitude modulation ( B ) was then used to extract the L / R ratios for each metabolite in the stroked region and contralateral hemisphere. Apparent metabolic T 1 measurements Apparent T 1 s were measured in both ipsi- and contralateral hemispheres of rats 3 h post ischaemia by applying a progressive saturation filter that entailed 16 dummy scans and 48 signal averages for TRs ranging between 0.7 and 7.1 s. These TRs were randomized to avoid any potential consistent effects. The data were then fit to the classic T 1 exponential buildup curves: M (TR) = M 0 [1−exp(−TR/ T 1 )]+y 0 . Apparent metabolic T 2 measurements Apparent T 2 s were measured in both ipsi- and contralateral hemispheres of rats 24 h post ischaemia by increasing the effective TE of the measurements, that is, by varying in an equidistant fashion the refocusing pulse separation (denoted under ‘Mechanism’ in Fig. 1 ) using a long TR of 6.5 s. Eight dummy scans and 16 signal averages were used for TEs ranging between 54 and 250 ms. TEs were randomized to avoid any potential systematic errors. The data was then fit to a classic T 2 exponential decay: M(TE) = M 0 [exp(−TE/ T 2 )]. How to cite this article: Shemesh, N. et al . Metabolic properties in stroked rats revealed by relaxation-enhanced magnetic resonance spectroscopy at ultrahigh fields. Nat. Commun. 5:4958 doi: 10.1038/ncomms5958 (2014).